In situ identification of the metallic state of Ag nanoclusters in oxidative dispersion 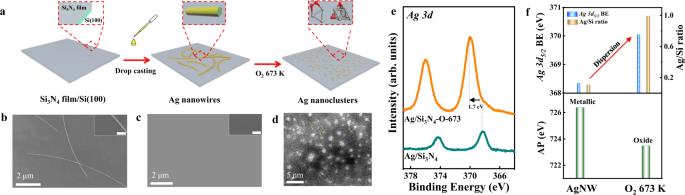Fig. 1: Oxidative dispersion of AgNWs. aScheme for the preparation of AgNWs onto Si3N4(Ag/Si3N4) and the subsequent oxidation treatment (Ag/Si3N4-O-673).b,cSEM images of Ag/Si3N4and Ag/Si3N4-O-673 samples. The scale bar in the insets is 200 nm.dHAADF-STEM image of Ag/Si3N4-O-673.eXPS Ag 3dspectra andfAg 3d5/2BE shift, Ag/Si ratio, and Auger parameter deduced from quasi in situ XPS data of Ag/Si3N4and Ag/Si3N4-O-673 samples. Oxidative dispersion has been widely used in regeneration of sintered metal catalysts and fabrication of single atom catalysts, which is attributed to an oxidation-induced dispersion mechanism. However, the interplay of gas-metal-support interaction in the dispersion processes, especially the gas-metal interaction has not been well illustrated. Here, we show dynamic dispersion of silver nanostructures on silicon nitride surface under reducing/oxidizing conditions and during carbon monoxide oxidation reaction. Utilizing environmental scanning (transmission) electron microscopy and near-ambient pressure photoelectron spectroscopy/photoemission electron microscopy, we unravel a new adsorption-induced dispersion mechanism in such a typical oxidative dispersion process. The strong gas-metal interaction achieved by chemisorption of oxygen on nearly-metallic silver nanoclusters is the internal driving force for dispersion. In situ observations show that the dispersed nearly-metallic silver nanoclusters are oxidized upon cooling in oxygen atmosphere, which could mislead to the understanding of oxidation-induced dispersion. We further understand the oxidative dispersion mechanism from the view of dynamic equilibrium taking temperature and gas pressure into account, which should be applied to many other metals such as gold, copper, palladium, etc. and other reaction conditions. Sintering is a longstanding problem in heterogeneous catalysis leading to deactivation after the long-term operation at high temperatures [1] , [2] , [3] . Many regeneration methods are developed to redisperse the sintered metal catalysts, such as oxidation–reduction, chlorination–oxychlorination, thermal treatment with halohydrocarbons, etc [2] , [4] , [5] , [6] . Among those, oxidative dispersion is one widely adopted process for the regeneration of used industrial catalysts [6] , [7] , [8] , [9] , [10] , [11] . It has been shown that sintered metal catalysts can break apart into highly dispersed oxide segments during oxidation and are then reactivated by reduction, yielding metal nanoclusters with restored activity [4] . Beyond catalyst regeneration, oxidative dispersion has recently been employed as one important route to fabricate single-atom catalysts (SACs) and oxidation treatment of supported metal catalysts in the oxidative atmosphere such as air, O 2 , and water vapor produces SACs of Pt, Pd, Rh, Ag, etc [12] , [13] , [14] , [15] , [16] , [17] , [18] . Hence, oxidative dispersion is of paramount importance for the fabrication and regeneration of highly/atomically dispersed catalysts with remarkable activity. Dispersion under oxidizing conditions is a common phenomenon reported in catalysts of Rh/CeO 2 , Pt/CHA(siliceous chabazite), Ru/CeO 2 , Ag/MnO x , Pt/FeO x , etc [6] , [12] , [13] , [19] , [20] . The consensus on the oxidative dispersion process includes the formation of mobile metal oxide species from large metal particles and capture of these species on the support surface, which are regarded as the most crucial steps in the so-called oxidation-induced dispersion mechanism as revealed by in situ electron microscopy and/or in situ spectroscopy [21] , [22] , [23] , [24] , [25] , [26] , [27] , [28] . For example, Nagai et al. ascribed the redispersion of Pt nanoparticles to the formation of Pt oxide species as observed in O 2 at 873 K by in situ X-ray absorption spectroscopy (XAS) [22] . Nevertheless, the underlying mechanism yet needs to be fully depicted. It is well known that the oxidation of metals is strongly dependent on both oxidant partial pressure and temperature. The high temperature applied in catalyst treatments, in general, does not favor the oxide formation, particularly for metals with small heat of formation of an oxide such as Au, Ag, Pd, etc [29] , [30] , [31] . Thus, more detailed investigation by in situ characterization is highly demanded in order to provide new and deep insights into the dynamic mechanism for the oxidative dispersion of supported metal catalysts. In this work, we performed a state-of-the-art study for the dynamic dispersion of Ag aggregates i.e., nanowires (NWs) and nanoparticles (NPs) supported on Si 3 N 4 surfaces upon heating in O 2 using a combination of ex situ, quasi in situ, and in situ characterization techniques including near-ambient pressure XPS (NAP-XPS), near-ambient pressure photoemission electron microscopy (NAP-PEEM), and environmental scanning (transmission) electron microscopy (ESEM/ESTEM). The oxidative dispersion of Ag aggregates has been unambiguously observed, which occurs via the formation of mobile metallic Ag nanoclusters rather than Ag oxide species, and remarkably enhances their catalytic reactivity in CO oxidation. Chemisorption of oxygen from mbar O 2 atmosphere is an essential driving force for the dispersion of nearly-metallic Ag nanoclusters under in situ conditions, verified by both experimental evidence and density functional theory (DFT) calculations. The dynamic dispersion of Ag during the reaction and its correlation to the catalytic reactivity is further demonstrated for CO oxidation reaction. Ex situ characterization of oxidation-induced dispersion of AgNWs Well-defined AgNWs [32] were drop-casted onto a Si 3 N 4 thin film (50 nm thick) grown on a Si(100) wafer, denoted as Ag/Si 3 N 4 (see “Methods” and Fig. 1a ). The as-prepared AgNWs (Fig. 1b ) show an average length of 20 μm with 80 nm in diameter. Thermal treatment in 1 mbar O 2 at 673 K results in the dispersion of all AgNWs into ultra-small Ag clusters on the Si 3 N 4 surface (denoted as Ag/Si 3 N 4 -O-673), rather than sintered aggregates. The small size makes them nearly invisible under SEM imaging as shown by Fig. 1c . High angle annular dark-field (HAADF)-STEM imaging further reveals the highly dispersed sub-nm Ag nanoclusters (Ag n ) with a significant number of atomic clusters and single atoms (marked by yellow arrows in Fig. 1d and supplementary Fig. 1 ). Fig. 1: Oxidative dispersion of AgNWs. a Scheme for the preparation of AgNWs onto Si 3 N 4 (Ag/Si 3 N 4 ) and the subsequent oxidation treatment (Ag/Si 3 N 4 -O-673). b , c SEM images of Ag/Si 3 N 4 and Ag/Si 3 N 4 -O-673 samples. 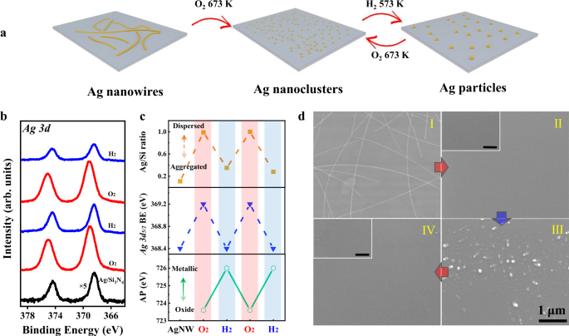Fig. 2: Reversible oscillation of Ag dispersion during redox cycles. aSchemes of redox cycles of Ag aggregates on Si3N4.bQuasi in situ XPS Ag 3dspectra of Ag nanostructures on Si3N4during redox cycles.cOscillation of Ag/Si ratio, Ag 3d5/2BE, and Auger parameter during O2/H2redox cycles.dEx situ SEM images of Ag/Si3N4sample upon repeated O2/H2redox treatment. The scale bar in the insets is 500 nm. I: pristine Ag/Si3N4sample; II: oxidation in 1 bar O2at 673 K; III: subsequent reduction in 0.1 bar H2at 573 K; IV: re-oxidation in 1 bar O2at 673 K. All XPS spectra were collected at room temperature. The scale bar in the insets is 200 nm. d HAADF-STEM image of Ag/Si 3 N 4 -O-673. e XPS Ag 3 d spectra and f Ag 3 d 5/2 BE shift, Ag/Si ratio, and Auger parameter deduced from quasi in situ XPS data of Ag/Si 3 N 4 and Ag/Si 3 N 4 -O-673 samples. Full size image Measured by quasi in situ XPS (Fig. 1e ), the pristine Ag/Si 3 N 4 surface shows Ag 3 d 5/2 binding energy (BE) of 368.3 eV which is characteristic of metallic silver [33] , whereas the Ag/Si 3 N 4 -O-673 sample presents a significant upshift of Ag 3 d 5/2 by +1.7 eV to 370.0 eV. Both Si 2 p and N 1 s spectra of the two samples remain unchanged (Supplementary Fig. 2 ), suggesting the high stability of the Si 3 N 4 film under the treatment condition. It is well known that Ag oxides usually have a similar or even lower Ag 3 d BE compared to Ag metal [12] . Therefore, the upshift of Ag 3 d BE in Ag/Si 3 N 4 -O-673 is not caused by the change of oxidation state, but more likely due to size effect [34] , [35] . It has been validated that the screening of core holes in ultra-small metal nanoclusters becomes limited which results in an upshift of core-level BEs [36] , [37] , [38] , [39] . Hence, the upshift of Ag 3 d BE is ascribed to the decreasing size of Ag aggregates from micrometer to sub-nanometer. Meanwhile, considering the surface sensitivity of XPS, Ag 3 d peak intensity of the Ag/Si 3 N 4 -O-673 sample also increases drastically, reflecting the gain of Ag surface area (surface-to-bulk ratio) during the transformation of AgNWs to highly dispersed Ag nanoclusters. To quantify, the peak area ratio of Ag 3 d 5/2 to Si 2 p (denoted as Ag/Si ratio) was derived and used as a representative for the dispersion degree of Ag nanostructures on Si 3 N 4 . As illustrated in Fig. 1f , both Ag/Si ratio and Ag 3 d 5/2 BE reflect the Ag dispersion degree for a given coverage (referred to Ag loadings on Si 3 N 4 substrate), suggesting the high dispersion of AgNWs after the O 2 treatment as proved by the SEM/STEM results (Fig. 1b–d ). Regarding the oxidation state of silver, it is unable to distinguish oxide or metallic state using XPS core-levels [12] , [33] . Alternatively, Auger Parameters (AP, α) (see the description of Auger parameter in the Supplementary Discussion ) defined as the sums of Auger kinetic energy (KE) and photoelectron BE are often used to identify the chemical state of elements including Cu, Ag, Zn, etc [37] , [40] , [41] . Auger spectra of Ag MNN are shown in supplementary Fig. 2 , and the sums of Ag 3 d 5/2 BE and Ag MNN KE were given in Fig. 1f . AP value for pristine Ag/Si 3 N 4 is about 726.4 eV as characteristic for metallic Ag [12] , [40] , while that of Ag/Si 3 N 4 -O-673 shows a lower value of 723.6 eV reflecting its nature of Ag oxides (e.g., Ag 2 O) [12] after the O 2 treatment. Overall, we can thus establish a criterion by using Ag/Si ratio and Ag 3 d 5/2 BE as indications for Ag dispersion degree, and AP value to describe the oxidation state. To further validate the universality of this dynamic dispersion of Ag on different supports, we have performed additional experiments on a variety of oxides including SiO 2 /Si(100), Al 2 O 3 (0001), and SrTiO 3 (110) substrates. The upshift of Ag 3 d BE and the increase in the Ag 3 d peak intensity were observed on all the substrates (supplementary Fig. 3 ), which is similar to that on the Si 3 N 4 surface ( Supplementary Discussion ). Reversible oscillation of Ag dispersion upon cyclic oxidation–reduction treatments Cyclic oxidation–reduction treatments (Fig. 2a ) were performed to investigate the dispersion-aggregation of Ag nanostructures in an alternative O 2 and H 2 atmosphere. Quasi in situ Ag 3 d XPS spectra (Fig. 2b ) and Ag MNN Auger spectra (supplementary Fig. 4 ) as well as ex situ SEM images (Fig. 2d ) reveal good reversibility of Ag dispersion upon the oxidation–reduction cycles. The deduced Ag/Si ratio, Ag 3 d 5/2 BE, and AP values are presented in Fig. 2c , and an oscillation of Ag dispersion and oxidation states is clearly demonstrated. After the first oxidation treatment (1 bar O 2 at 673 K for 1 h), a highly dispersed state of silver oxide (AgO x ) nanoclusters was identified at room temperature. The increasing Ag/Si ratio and the upshift of Ag 3 d 5/2 BE are characteristic of the high dispersion state, and the lower AP value infers its oxide nature. The ultra-small AgO x nanoclusters are likely below 1 nm making them invisible under SEM imaging (Fig. 2d, II ). Fig. 2: Reversible oscillation of Ag dispersion during redox cycles. a Schemes of redox cycles of Ag aggregates on Si 3 N 4 . b Quasi in situ XPS Ag 3 d spectra of Ag nanostructures on Si 3 N 4 during redox cycles. c Oscillation of Ag/Si ratio, Ag 3 d 5/2 BE, and Auger parameter during O 2 /H 2 redox cycles. d Ex situ SEM images of Ag/Si 3 N 4 sample upon repeated O 2 /H 2 redox treatment. The scale bar in the insets is 500 nm. I: pristine Ag/Si 3 N 4 sample; II: oxidation in 1 bar O 2 at 673 K; III: subsequent reduction in 0.1 bar H 2 at 573 K; IV: re-oxidation in 1 bar O 2 at 673 K. All XPS spectra were collected at room temperature. Full size image The subsequent reduction (0.1 bar H 2 at 573 K for 1 h) leads to strong sintering as indicated by the decreasing Ag/Si ratio and the downshift of Ag 3 d 5/2 BE. The reduction to metallic Ag state is verified by the higher AP value. The sintered Ag metal particles show a size range of 10–200 nm measured by SEM (Fig. 2d, III ). The re-oxidation (Fig. 2d, IV ) can repeatedly disassemble the aggregated Ag particles into ultra-small AgO x clusters. The results indicate that the oxidative dispersion behavior does not rely on the morphology of Ag aggregates, no matter of NWs or NPs. The second reduction shows a good reproducibility yielding metallic Ag aggregates after the H 2 treatment. The observed reversible oscillation of Ag dispersion during redox cycles opens the feasibility to control the dispersion of Ag catalysts via oxidation/reduction pretreatments. Solely based on quasi in situ XPS and ex situ EM results, we can demonstrate oxidative dispersion of μm-scale metallic AgNWs into sub-nm AgO x clusters through 1 mbar–1 bar O 2 treatment at 673 K. These ex situ observations are seemingly in line with the previous understanding for the oxidation-induced dispersion mechanism. However, our in situ experiments disproved this “common sense” and further revealed the role of oxygen atmosphere as discussed in the following section. In situ observation of oxidative dispersion In order to elucidate the dynamic process of the Ag dispersion, we performed NAP-XPS studies on Ag/Si 3 N 4 in 1 mbar O 2 during heating from 300 to 700 K (Fig. 3a ). No obvious change in XPS Ag 3 d spectra was observed in a range of 300–600 K. The slight increase of Ag 3 d peak intensity is ascribed to the removal of carbon residuals on the sample surface (see C 1 s spectra in Supplementary Fig. 5 ). Further increasing temperature to 700 K results in a sharp increase of Ag/Si ratio along with a prominent BE shift of Ag 3 d 5/2 from 368.1 to 370.2 eV (Fig. 3b ), which serves as a clear indication for the dispersion of AgNWs into small Ag clusters. Fig. 3: In situ observation of dynamic dispersion of AgNWs in 1 mbar O 2 . a NAP-XPS Ag 3 d spectra and b Ag 3 d 5/2 BE and Ag/Si ratio of Ag/Si 3 N 4 sample upon heating from 300 to 700 K in 1 mbar O 2 . c In situ visualization of dynamic dispersion of AgNWs at 673 K in 1 mbar O 2 by ESEM. Full size image Direct imaging of dynamic dispersion of AgNWs was performed in situ using ESEM in 1 mbar O 2 at 673 K (Fig. 3c and Supplementary Video 1 ). Initially, intact AgNWs were observed on Si 3 N 4 surface at t = 0 min. Subsequently, the dispersion of AgNWs occurs at t = 15 min, along with the spread-out of Ag nanoclusters (<1 nm) to the free substrate surface resulting in the invisibility of Ag under SEM ( t = 30 min). The dispersion sustains with increasing time and eventually leads to a nearly complete disappearance of AgNWs at t = 45 min. Similarly, the dispersion process was further confirmed by NAP-PEEM [42] (Supplementary Fig. 6 ), which was conducted at 873 K in O 2 ambience up to 0.1 mbar. The bright contrast of AgNWs in PEEM images is due to the low surface work function of metallic Ag [43] . When exposed to O 2 , part of NW was observed to become dark and the darkening gradually extended to the whole NW (Supplementary Fig. 6 ), indicating the diffusion of silver atoms from NWs to the bared substrate surface [43] . Both in situ spectroscopic and microscopic measurements provide a clear picture of the high dispersion of AgNWs at elevated temperatures driven by O 2 . Role of oxygen: surface oxygen adsorption vs. bulk oxidation It has been well accepted that bulk oxidation with a high oxidation degree is the key step in the dispersion of metal particles in O 2 at elevated temperatures [6] , [11] , [14] , [20] , [44] , [45] . However, whether bulk oxidation is necessary for oxidative dispersion of supported metal catalysts still requires to be validated. To this end, we performed NAP-XPS studies of AgNWs on Si 3 N 4 under different conditions in the following sequence: I, pristine Ag/Si 3 N 4 under UHV at room temperature; II, 1 mbar O 2 at 700 K; III, UHV at 700 K; IV, 1 mbar O 2 at 700 K; V, 1 mbar O 2 at 450 K; VI, 1 mbar O 2 at 300 K. All XPS core-level and Auger peaks were measured in situ at the treatment temperatures and under the certain environments as presented in Fig. 4a, b , and the corresponding Ag/Si ratios and AP values were displayed in Fig. 4c . Fig. 4: Evolution of Ag during in situ experimental conditions. NAP-XPS results of Ag 3 d spectra ( a ) and Ag MNN Auger spectra ( b ) of Ag/Si 3 N 4 under in situ experimental conditions. I: Ag/Si 3 N 4 ; II: 1 mbar O 2 at 700 K; III: UHV (1 × 10 − 6 mbar) at 700 K; IV: 1 mbar O 2 at 700 K; V: cooling to 450 K in 1 mbar O 2 ; VI: cooling to 300 K in 1 mbar O 2 . c Deduced Auger parameter and Ag/Si ratio from NAP-XPS data, and temperature profile for in situ experimental conditions. d The relative formation energy of Ag 3 cluster and Ag 8 cluster based on the Ag particle under considering different influencing factors. Full size image The results show that calcinating at 700 K in 1 mbar O 2 (condition II) leads to a significant increase in Ag/Si ratio indicating the dispersion of AgNWs. The AP value remains at 726.0 eV (errors in the range from −0.3 to 0.3 eV due to the broad Ag Auger peaks) that strongly infers a metallic state of dispersed Ag species under in situ condition (700 K, 1 mbar O 2 ). This can be rationalized by the Ag-O phase diagram showing that oxides are prone to decompose into metallic phase at 700 K in 1 mbar O 2 [29] . It suggests that the formation of bulk oxide with a high oxidation degree is not necessary for stabilizing highly dispersed metallic species. To our best knowledge, it is the first evidence that elucidates the dispersion in the form of nearly-metallic clusters rather than bulk oxide (with a high oxidation degree) during oxidative dispersion. A similar metallic state of dispersed Ag species was also observed on the SiO 2 /Si(100) surface in O 2 at elevated temperatures, verifying a universal phenomenon for SiO 2 and other oxides (Supplementary Fig. 7 ). After removing mbar O 2 to UHV condition (condition III), sintering of dispersed Ag nanoclusters occurs, forming aggregated particles as indicated by the smaller Ag/Si ratio. In absence of O 2 atmosphere, the gain of surface energy favors the sintering of Ag metal particles, e.g., Ostwald ripening, which suggests that adsorbed oxygen species from the O 2 atmosphere play a critical role in stabilizing highly dispersed Ag nanoclusters. Previous surface science studies on Ag foils and Ag single crystals indicated that adsorbed oxygen species are formed at Ag surfaces at high temperature in O 2 [46] , [47] , [48] , rather than producing bulk oxides (Ag 2 O). Hence, chemisorption of oxygen on metallic Ag surface is suggested as a possible driving force for the dynamic dispersion of AgNWs/aggregates into sub-nm Ag clusters during the oxidative dispersion. The reversibility of adsorption-driven dispersion-aggregation is further proved by re-exposure of the sintered Ag aggregates to O 2 at 700 K (Fig. 4c IV ). During the entire process, nearly-metallic state of Ag is preserved as indicated by the constant AP value of 726.0 eV for all four states (I, II, III, and IV). The cooling process of highly dispersed Ag nanoclusters in 1 mbar O 2 from 700 to 300 K was further investigated by changing from condition IV to VI. Cooling down in 1 mbar O 2 to 450 and 300 K results in a prominent downshift of AP value to 724.6 eV suggesting the formation of AgO x upon cooling in O 2 (Fig. 4c, IV–VI ). Meanwhile, the constant Ag/Si ratio (Fig. 4c, IV–VI ) reveals that the high dispersion of Ag nanoclusters is still preserved at low temperatures. Therefore, we can depict an overall picture of dynamic dispersion of AgNWs in 1 mbar O 2 by two independent processes: (1) surface oxygen adsorption-driven dispersion of AgNWs to Ag nanoclusters at 700 K, and (2) oxidation of readily dispersed Ag nanoclusters to bulk-like AgO x nanoclusters with a high oxidation degree during cooling to 300 K. Our in situ characterizations allow to conclude that the chemisorption of oxygen on metallic silver is the driving force for Ag dispersion whereas the bulk oxide with a high oxidation degree is only the result upon cooling in O 2 . DFT study in oxidative dispersion mechanism We proposed a DFT-based model to understand the O 2 adsorption-induced dispersion. The equation for this model is described in the “Methods” section (Eq. ( 1 )). The competing mechanism among cohesive energy ( E coh , metal-metal interaction), adhesion energy ( E adh , metal-support interaction), and gas adsorption energy ( E ads , metal-gas interaction) has been considered thoroughly, the sum of which constitutes the formation energy of the NP/cluster on the support under in situ conditions. The difference of the averaged formation energy/atom between the sintered NP and the dispersed cluster \(({\Delta}E_{\mathrm{for}})\) , thus determines the dynamic dispersion, and the positive \({\Delta}E_{\mathrm{for}}\) favors the dispersion. Considering the very large average sizes of the sintered NPs in this work (over 100 nm), we used the cohesive energy/atom of bulk Ag \((E_{\mathrm{{coh}}}^{\mathrm{{bulk}}})\) to represent the NP’s E coh (set α in Eq. ( 1 ) to be 12), which is −2.79 eV in our calculation. Ag 3 and Ag 8 clusters were used as the models for the cluster calculations, the \(E_{\mathrm{{coh}}}^{\mathrm{{clu}}}\) of which are calculated to be −1.21 and −1.86 eV, respectively. Thus, in their freestanding states, ΔE for are −1.58 and −0.93 eV, respectively (Fig. 4d ). When supported on the surface, the averaged E adh /atom of the sintered NP is neglectable because the ratio of the interface to volume for such a large particle is very small. On the other hand, the averaged E adh /atom of Ag 3 and Ag 8 clusters are calculated to be −0.96 and −0.56 eV on the supported Si 3 N 4 (0001) surface (Supplementary Figs. 8 , 9 ), respectively. Consequently, \({\Delta}E_{\mathrm{for}}\) becomes −0.62 and −0.37 eV, respectively, which are still negative, suggesting that the addition of metal-support interaction is insufficient to disperse Ag NPs into nanoclusters. This thus explains the aggregated state of Ag particles under UHV condition during in situ experiments in Fig. 4c, III when O 2 is removed from the atmosphere. When O 2 adsorption is involved, the reaction condition effects (temperature and gas pressure) are considered through the calculation of gas adsorption coverage θ i by using a DFT-based thermodynamic adsorption isotherm described in the methods section [49] , [50] , [51] . We used the gas coverage of O 2 on three low-index surfaces ( \(\theta ^{111},\;\theta ^{110},\;\theta ^{100}\) ) to estimate θ i of the sintered NP because a nanosized Ag particle is normally composed of these surfaces (supplementary Fig. 10 ). The results show that O 2 barely adsorbs on the three surfaces at 673 K even with an O 2 pressure of 1 bar due to the small adsorption energies ( \(E_{\mathrm{ads}}^{111} = - 0.40\) eV, \(E_{\mathrm{ads}}^{110} = - 0.38\) eV, \(E_{\mathrm{ads}}^{100} = - 0.76\) eV). On the contrary, associative O 2 and dissociative O atoms adsorb stably at the Ag 3 -Si 3 N 4 ( \(E_{\mathrm{ads}}^{\mathrm{clu}} = - 2.24\;{\mathrm{eV}}\) ) and Ag 8 -Si 3 N 4 ( \(E_{\mathrm{ads}}^{\mathrm{clu}} = - 3.97\;{\mathrm{eV}}\) ) interfaces, which leads to \(\theta ^{\mathrm{clu}} = 1\) for both models at 673 K under either 1 mbar O 2 or 1 bar O 2 . The averaged \(E_{\mathrm{ads}}^{\mathrm{clu}}\) /atom is −0.75 and −0.50 eV, respectively, which eventually makes \({\Delta}E_{\mathrm{for}}\) positive (0.13 eV for both models, Fig. 4d ). Compared to the sintered NP, dispersed nanoclusters have more contact with the support surface and the O 2 gas environment. Neither the support effect nor the O 2 adsorption could cause the dispersion of Ag NPs observed in our experiments, but the combined effects are enough to pry the lever. Dynamic dispersion during CO oxidation reaction The dynamic dispersion of Ag nanostructures during the reaction was further verified for CO oxidation [11] , [48] , [52] , [53] , [54] and the impact on their catalytic activity was investigated. In situ ESEM images (Fig. 5a ) show the dynamic dispersion of AgNWs under reaction conditions of 5% CO/95% O 2 at 1 mbar. The dispersion of AgNWs initially occurs at 623 K and reaches a highly dispersed state at 673 K. The highly dispersed Ag nanoclusters remain in the reaction gases during cooling. The catalytic test was further performed in a home-built flow reactor with an online mass spectrometer to the outlet for product analysis (see Supplementary Methods ). The reactivity for catalytic CO oxidation reaction was present in Fig. 5b and Supplementary Fig. 11 , and a hysteresis phenomenon was clearly identified upon heating and cooling cycle, as the result of the dynamic structure evolution of Ag during the reaction. The highly dispersed Ag nanoclusters formed during reaction exhibit an enhanced activity especially at low temperature, higher than the initial state of AgNWs upon heating. A similar reactivity at 623 K indicates the structural transformation from NWs to nanoclusters which is consistent with the in situ ESEM observations. The time-on-stream stability test displayed in Fig. 5c further reveals excellent durability of the highly dispersed Ag/Si 3 N 4 catalyst under the reaction condition (at 673 K) up to 35 h (also see Supplementary Discussion ). Our results thus prove the long-term stability of dispersed nearly-metallic Ag nanoclusters in O 2 -rich reaction environments, and opens up a new route for the fabrication of highly dispersed catalysts during the reaction. Fig. 5: Dynamic Ag dispersion during CO oxidation. a In situ ESEM imaging of dynamic Ag dispersion during the reaction in 5% CO/95% O 2 at 1 mbar. The scale bar is 4 μm for all ESEM images. b The CO conversion for Ag/Si 3 N 4 upon the heating and cooling cycle. c The time-on-stream stability test of Ag/Si 3 N 4 under the reaction condition at 673 K. Full size image Dynamic dispersion of AgNWs into sub-nm Ag clusters on Si 3 N 4 surface has been observed using combined ex situ and in situ characterization techniques. By altering oxidizing/reducing treatments, we can reversibly switch between highly dispersed Ag nanoclusters (0.7 nm) and aggregated Ag particles (20–100 nm). Based on ex situ characterizations, we readily observed the formation of dispersed silver oxides at room temperature after the high-temperature treatment in O 2 , which is in line with the commonly accepted “oxidation dispersion” scenario. 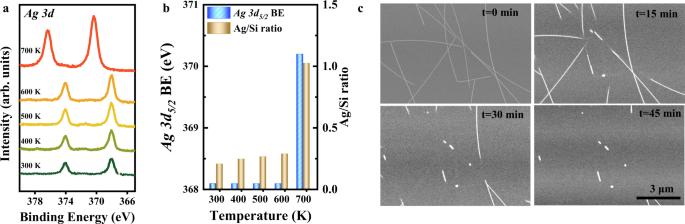Fig. 3: In situ observation of dynamic dispersion of AgNWs in 1 mbar O2. aNAP-XPS Ag 3dspectra andbAg 3d5/2BE and Ag/Si ratio of Ag/Si3N4sample upon heating from 300 to 700 K in 1 mbar O2.cIn situ visualization of dynamic dispersion of AgNWs at 673 K in 1 mbar O2by ESEM. However, as Fig. 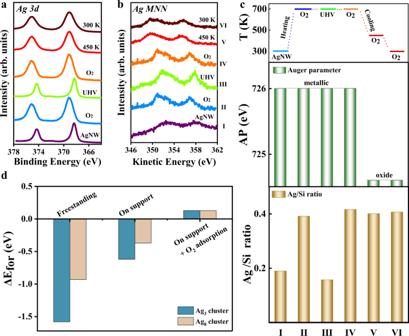Fig. 4: Evolution of Ag during in situ experimental conditions. NAP-XPS results of Ag 3dspectra (a) and Ag MNN Auger spectra (b) of Ag/Si3N4under in situ experimental conditions. I: Ag/Si3N4; II: 1 mbar O2at 700 K; III: UHV (1 × 10−6mbar) at 700 K; IV: 1 mbar O2at 700 K; V: cooling to 450 K in 1 mbar O2; VI: cooling to 300 K in 1 mbar O2.cDeduced Auger parameter and Ag/Si ratio from NAP-XPS data, and temperature profile for in situ experimental conditions.dThe relative formation energy of Ag3cluster and Ag8cluster based on the Ag particle under considering different influencing factors. 6 summarized, our in situ studies directly demonstrated a transitional state of nearly-metallic Ag during dispersion that overturn this common concept and depict an overall scenario of dynamic dispersion under O 2 environment consisting of oxygen adsorption-induced dispersion of Ag in a nearly-metallic state at 700 K and oxidation of readily dispersed Ag nanoclusters to Ag oxide nanoclusters during cooling to 300 K. We provide solid evidence for the fact that formation of bulk oxide with a high oxidation degree is not necessary in oxidative dispersion, but a result during cooling in O 2 . Chemisorption of oxygen on nearly-metallic Ag rather than bulk oxidation is proved as the driving force to disperse Ag aggregates and stabilize ultra-small Ag clusters under in situ conditions. Correctly understanding the role of O 2 environment played in oxidative dispersion is of great significance in predicting and controlling the dynamics of dispersion/redispersion of supported metal catalysts under reaction conditions. It also opens up a new route to stabilize metal nanoclusters in a realistic reaction atmosphere, and benefits the fabrication of highly/atomically dispersed catalyst during reaction. Fig. 6: Dynamic evolution of Ag during oxidative dispersion. The description of adsorption-driven dispersion mechanism rather than oxidation-induced dispersion mechanism. Full size image Sample preparation and treatment AgNWs were synthesized via a polyol method and then purified by a novel dynamic agitation-induced centrifugal filtration [32] . Si 3 N 4 film (50-nm thick) grown on Si(100) single crystals were purchased from Prmat (Shanghai) Technology Co., Ltd. The inert Si 3 N 4 films are nearly free of surface defects [55] and remain stable under reaction conditions (see Supplementary Discussion ). AgNWs in ethanol solution were drop-casted onto the Si 3 N 4 substrate (denoted as Ag/Si 3 N 4 ). We prepared three kinds of samples with different Ag densities (high, medium, and low). To acquire strong Auger spectra, samples with high NW density were used and shown in Fig. 4 . Samples with medium AgNW density were used to get an obvious change of Ag/Si ratio during various treatments, also to make XPS peak intensity strong enough, shown in Figs. 1 – 3 . Samples with low density were used in electron microscopy (SEM, STEM, PEEM) to observe the process easily. The effect of surface concentration in our experiments was excluded by SEM results (Supplementary Fig. 16 ). Ex situ treatments were performed in 1 mbar O 2 , 1 bar O 2 , or 100 mbar H 2 at elevated temperatures in a high-pressure reactor (SPECS, HPC-20) (denoted as Ag/Si 3 N 4 - x - y , x is the atmosphere and y is the temperature). Scanning transmission electron microscopy AC-STEM was performed on a JEM ARM200F (JEOL, Japan), equipped with a thermal-field emission gun and a Cs-corrector. The microscope was operated at 80 kV to minimize the beam damage. For the high angle annular dark-field (HAADF) imaging, the convergence angle of ~23 mrad and collection angle range of 68–174 mrad were adapted for the incoherent atomic number imaging. In situ NAP-XPS Surface chemistry of Ag/Si 3 N 4 was characterized in a lab-based near-ambient pressure X-ray photoelectron spectroscopy (SPECS EnviroESCA). Spectra were obtained using monochromatic Al Kα irradiation (1486.7 eV) of an Al anode operated at 50 W. A pass energy of 40 eV with a step of 0.05 eV and a dwell time of 0.1 s were typically used for acquiring the core-level spectra. 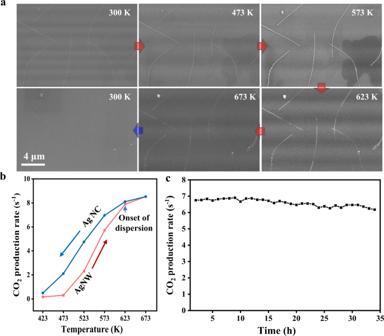Fig. 5: Dynamic Ag dispersion during CO oxidation. aIn situ ESEM imaging of dynamic Ag dispersion during the reaction in 5% CO/95% O2at 1 mbar. The scale bar is 4 μm for all ESEM images.bThe CO conversion for Ag/Si3N4upon the heating and cooling cycle.cThe time-on-stream stability test of Ag/Si3N4under the reaction condition at 673 K. 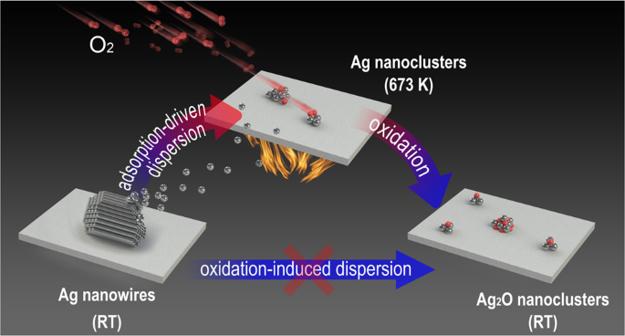Fig. 6: Dynamic evolution of Ag during oxidative dispersion. The description of adsorption-driven dispersion mechanism rather than oxidation-induced dispersion mechanism. Quasi in situ XPS Quasi in situ XPS measurements were carried out with a spectrometer equipped with an Mg Kα X-ray source operated at 300 W. The background pressure was in the range of 10 −9 mbar. Ex situ treatments were performed in the high-pressure reactor (SPECS, HPC-20). After each treatment, the sample was transferred to the analysis chamber for XPS measurements without exposure to air. All quasi in situ XPS spectra were collected under UHV (10 −9 –10 − 10 mbar) at room temperature. In situ ESEM In situ SEM imaging was performed in a commercial ESEM (FEI Quanta 650) equipped with a commercial heating stage and a gas feeding unit. The accelerating voltage was 20 kV with an objective lens aperture of 30 μm. During heating, low magnification was used to locate the targeted area due to thermal drift, and high magnification imaging (×20,000) was conducted when the temperature is stable. In situ NAP-PEEM PEEM experiments were performed on a newly developed NAP-PEEM system, which enables high-resolution PEEM imaging in gases with pressures up to 1 mbar. A tunable deep ultraviolet (DUV) laser with wavelength between 175 and 210 nm was used as an excitation source. The sample was heated up by a specially design laser heater, and the sample temperature was measured by an infrared thermometer. The in situ PEEM imaging was conducted by first heating the sample to a specific temperature and then dosing O 2 with increasing pressures. Catalytic testing The sample was prepared by drop-casting of AgNWs onto Si 3 N 4 /Si(100) surfaces (10 mm × 10 mm) with a silver loading of 1 μg. The catalytic test was performed in a home-built cell reactor (setup details see Supplementary Methods ) in a gas flow of 10 ml/min 5% CO/95% O 2 at atmospheric pressure. The reaction product (CO 2 , m / z 44) was monitored by an online mass spectrometer (SRS RGA) to the outlet of the reactor. The cell reactor was repeatedly purged and flushed with the reaction gas for >6 h to achieve a clean background. All catalysts were pre-reduced in 5% H 2 at 100 °C for 30 min before catalytic measurements. Equation for the adsorption-induced dispersion model Equation ( 1 ) is the formula we used to estimate the energy difference per atom between a sintered NP and dispersed clusters on the support under the O 2 gas conditions. ΔE_for = α/12E_coh^bulk + ( E_adh^par/N_par + ∑_i = 1^N_surfθ ^iE_ads^i/N_par) - E_coh^clu - ( E_adh^clu/N_clu + θ ^cluE_ads^clu/N_clu)
 (1) The first term in Eq. ( 1 ) is the cohesive energy per atom of the sintered NP, in which \(E_{\mathrm{coh}}^{\mathrm{bulk}}\) is the cohesive energy of a bulk Ag atom, α represents for the average coordination number of a sintered NP, and 12 is the coordination number of bulk Ag. The support effect and the O 2 adsorption effect on the sintered NP are considered in the second term, in which \(E_{\mathrm{adh}}^{\mathrm{par}}\) is the adhesion energy of the NP on the support, θ i is the adsorption coverage of O 2 at the i th surface site, \(E_{\mathrm{ads}}^i\) is the corresponding adsorption energy, \(N_{\mathrm{surf}}\) is the number of surface sites, and \(N_{\mathrm{par}}\) is the number of atoms of the NP. The third term ( \(E_{\mathrm{coh}}^{\mathrm{clu}}\) ) is the cohesive energy of the dispersed cluster averaged to each atom. The support effect and the O 2 adsorption effect on the dispersed cluster are considered in the fourth term, in which \(E_{\mathrm{adh}}^{\mathrm{clu}}\) is the adhesion energy of the cluster on the support, \(\theta ^{\mathrm{clu}}\) is the adsorption possibility, \(E_{\mathrm{ads}}^{\mathrm{clu}}\) is the corresponding adsorption energy, and \(N_{\mathrm{clu}}\) is the number of atoms of the cluster. If the formation energy difference per atom \({\Delta}E_{\mathrm{for}}\) is larger than zero, the dispersion of the nanoclusters is preferred. The DFT settings can be found in the Supplementary Information . DFT-based thermodynamic adsorption isotherm The O 2 coverage ( θ ) at a given adsorption site was described using the Langmuir adsorption isotherm. The formula is shown below, 
    θ = PK/(1 + PK)
 (2) where P is the gas pressure, K is the equilibrium constant calculated as below: 
    K = exp(  - ΔG/RT) = exp(  - E_ads - T( S_ads - S_gas)/RT)
 (3) where R is the gas constant, T is the temperature, \(E_{\mathrm{ads}}\) is the gas adsorption energy obtained from DFT calculations, \(S_{\mathrm{ads}}\) and \(S_{\mathrm{gas}}\) are the entropy of adsorbed O 2 and gas-phase O 2 , respectively. In this work, \(S_{\mathrm{ads}}\) was set to be 0 and \(S_{\mathrm{gas}}\) was obtained from the thermodynamic table ( https://www.nist.gov/srd ).